PKA catalytic subunit mutations in adrenocortical Cushing’s adenoma impair association with the regulatory subunit We recently identified a high prevalence of mutations affecting the catalytic (Cα) subunit of protein kinase A (PKA) in cortisol-secreting adrenocortical adenomas. The two identified mutations (Leu206Arg and Leu199_Cys200insTrp) are associated with increased PKA catalytic activity, but the underlying mechanisms are highly controversial. Here we utilize a combination of biochemical and optical assays, including fluorescence resonance energy transfer in living cells, to analyze the consequences of the two mutations with respect to the formation of the PKA holoenzyme and its regulation by cAMP. Our results indicate that neither mutant can form a stable PKA complex, due to the location of the mutations at the interface between the catalytic and the regulatory subunits. We conclude that the two mutations cause high basal catalytic activity and lack of regulation by cAMP through interference of complex formation between the regulatory and the catalytic subunits of PKA. Protein kinase A (PKA) is the primary mediator of cyclic AMP (cAMP) in eukaryotic cells and probably the best-studied protein kinase [1] . It consists of two regulatory (R) and two catalytic (C) subunits that assemble into a functional tetramer. In the holoenzyme, access to the active site cleft of the C subunit is prevented by interaction with an inhibitory sequence in the R subunit, which is tightly bound and serves as a tethered pseudosubstrate (RI subunits) or substrate (RII subunits) [1] . On binding of cAMP to two separate sites on each R subunit, the C subunits are released and become capable of phosphorylating Ser/Thr residues in a large number of target proteins [1] . Endocrine cells are under the strict control of hormones and local messengers that act primarily through G-protein-coupled receptors. Several of these receptors activate the cAMP/PKA pathway, leading in most cases to both increased hormone production and cell replication. Thus, somatic mutations causing constitutive activation of the cAMP/PKA pathway have been shown in several instances to be responsible for tumour formation and excessive hormone production, ultimately leading to endocrine disorders such as hyperthyroidism [2] , [3] or gigantism/acromegaly [4] , [5] . Moreover, germline-inactivating mutations in the PRKAR1A gene, coding for the PKA RIα subunit, have been linked to Carney complex, a rare syndrome characterized by excess of several hormones—most commonly cortisol excess (Cushing’s syndrome) due to the presence of multiple pigmented adrenal adenomas—as well as by cutaneous and neuronal tumours, skin and cardiac myxomas, and characteristic lesions of the skin and mucosae [6] . Similarly, mosaic, activating mutations of the gene coding for the Gα s protein ( GNAS1 , guanine nucleotide-binding protein, alpha-stimulating activity polypeptide 1) are responsible for the McCune–Albright syndrome, which is characterized by hormonal disorders, including in some cases cortisol excess due to adrenal hyperplasia [5] , [7] , [8] . Finally, mutations in PRKAR1A as well as in PDE11A and PDE8B , coding for two phosphodiesterases that are responsible for cAMP degradation, have also been associated with adrenal hyperplasia or unilateral cortisol-producing adenomas [9] , [10] , [11] , [12] . However, these mutations are found only in a small fraction of adrenal tumours. Recently, we identified a high prevalence of somatic mutations in PRKACA , coding for the Cα subunit of PKA, in a series of cortisol-secreting adrenal adenomas leading to Cushing’s syndrome [13] . The two identified mutations (c.617A>C, p.Leu206Arg and c.595_596insCAC, p.Leu199_Cys200insTrp) were present in the tumours but not in the surrounding normal adrenal tissue or in peripheral leucocytes. When expressed in cell lines, Cα subunits harbouring these mutations displayed normal catalytic activity, but were constitutively active as shown by the fact that their activity could no longer be suppressed by an excess of R subunits and was virtually not regulated by cAMP [13] . The same Leu206Arg mutation was very recently reported in similar studies by other groups [14] , [15] , [16] . These studies confirmed that this mutation causes increased PKA activity. However, there is considerable controversy regarding the underlying biochemical mechanism. Here we use a combination of biochemical and optical methods based on fluorescence resonance energy transfer (FRET) to clarify the mechanism of action of both PRKACA mutations associated with cortisol-secreting adrenal adenomas. The results indicate that these mutations interfere with the formation of a stable PKA holoenzyme both in vitro and in living cells, thus providing a molecular explanation for the constitutive activation of PKA caused by both mutations. In silico analysis of PRKACA mutations Both PRKACA mutations identified in cortisol-secreting adrenal adenomas (c.617A>C, p.Leu206Arg and c.595_596insCAC, p.Leu199_Cys200insTrp) affect amino acids in the so-called P+1 loop [1] that are positioned right at the interface between the R and C subunits ( Fig. 1a,b ). In particular, Leu206 is part of the active site cleft of the catalytic subunit and participates in the formation of a hydrophobic pocket, which is involved in substrate binding and recognition, as well as in the interaction with the inhibitory sequence of the R subunit [1] , [17] , [18] ( Fig. 1a ). On the basis of the known structure of the wild-type PKA holoenzyme [19] , we predict that substitution of Leu206 by a bulky and positively charged amino acid such as Arg could lead to direct steric hindrance between the side chain of this amino acid and that of both Val115 and Tyr228 in the R subunit ( Fig. 1c,d ). For the second mutation, which is more difficult to evaluate since it involves the insertion of an amino acid, it is noteworthy that Leu199 and Cys200 are located next to Thr198 in the so-called activation loop. The latter residue is phosphorylated after synthesis of the C subunit, which is required for full catalytic activity. Furthermore, these residues are located in a region of the C subunit that is oriented parallel to the inhibitory sequence, where residues Gly201 as well as Leu199 are involved in main-chain hydrogen bonding interactions with Val115 and Ala117 of the R subunit ( Fig. 1b ). Thus, the insertion of an additional residue, especially one with a very bulky side chain such as Trp, is also predicted to interfere with the interaction between the C and the R subunits. On the basis of these observations and the previous finding that both PKA Cα mutants are constitutively active despite the presence of an excess of R subunits and regardless of the intracellular concentration of cAMP [13] , we hypothesized that both mutations might interfere with the interaction between the C and R subunits, causing the C subunits to be free and, thus, active even in the absence of cAMP. 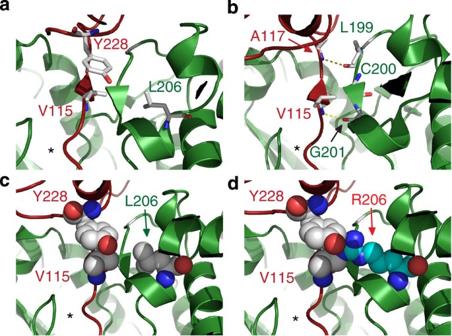Figure 1: Location of Leu206Arg and Leu199_Cys200insTrp mutations. (a–d) Zoomed in regions of the interface between the R (red) and C (green) subunits based on the structure of the mouse full-length tetrameric RIIβ(2):Cα(2) holoenzyme19(Protein Data Bank entry 3TNP). The inhibitory sequence is indicated by an asterisk (*). (a) Position of Leu206, shown in sticks. Val115 and Tyr228 in the R subunit are also depicted. (b) Position of residues Leu199 and Cys200, both shown as sticks. Gly201 in the C subunit as well as Val115 and Ala117 in the R subunit are also depicted. (c) Space-filling representation of Leu206, Val115 and Tyr228. (d)In silicoreplacement of Leu206 with Arg. The bulky and positively charged Arg side chain is predicted to clash with Val115 and Tyr228 in the R subunit, all shown in space-filling representation. Figure 1: Location of Leu206Arg and Leu199_Cys200insTrp mutations. ( a – d ) Zoomed in regions of the interface between the R (red) and C (green) subunits based on the structure of the mouse full-length tetrameric RIIβ(2):Cα(2) holoenzyme [19] (Protein Data Bank entry 3TNP). The inhibitory sequence is indicated by an asterisk (*). ( a ) Position of Leu206, shown in sticks. Val115 and Tyr228 in the R subunit are also depicted. ( b ) Position of residues Leu199 and Cys200, both shown as sticks. Gly201 in the C subunit as well as Val115 and Ala117 in the R subunit are also depicted. ( c ) Space-filling representation of Leu206, Val115 and Tyr228. ( d ) In silico replacement of Leu206 with Arg. The bulky and positively charged Arg side chain is predicted to clash with Val115 and Tyr228 in the R subunit, all shown in space-filling representation. Full size image Functional characterization of PKA Cα mutants in vitro As a first step to verify our hypothesis, we performed co-immunoprecipitation (co-IP) experiments investigating the basal association between PKA Cα mutants and R subunits. For this purpose, we transfected HEK293 cells with FLAG-tagged RIIβ and either wild-type or mutant Cα subunits at comparable expression levels. Using anti-FLAG antibodies, FLAG-tagged RIIβ was then immunoprecipitated from lysates of these cells and analysed for association with endogenous or exogenous Cα subunits by western blot analyses using an antibody directed against Cα. As expected, this resulted in a robust co-IP of the exogenously expressed wild-type Cα subunit ( Fig. 2 ). In contrast, only faint signals were detected in case of the Cα mutants, suggesting a much weaker interaction ( Fig. 2 ). The immunoprecipitation was specific as indicated by control experiments in which either the FLAG-tagged RIIβ subunit was omitted or the samples were mock precipitated ( Supplementary Fig. 1 ). 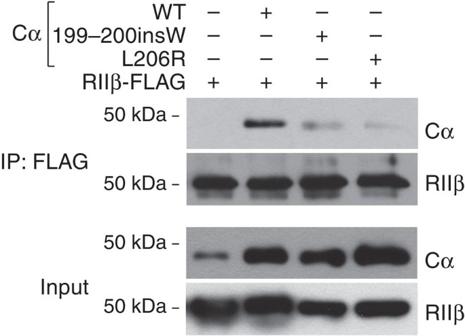Figure 2: Effect of Leu206Arg and Leu199_Cys200insTrp mutations on the association with R subunits analysed by co-IP. Cells were transfected with FLAG-tagged RIIβ (RIIβ-FLAG) and either wild-type (WT) or mutant Cα subunits. Shown are representative western blot analyses of Cα and RIIβ after FLAG-tagged RIIβ was immunoprecipitated with a FLAG-specific antibody (IP: FLAG). The western blot analyses in the lower part of the figure (input) control for expression levels of wild-type or mutant Cα and RIIβ. These analyses were repeated in at least six independent experiments with similar results. Figure 2: Effect of Leu206Arg and Leu199_Cys200insTrp mutations on the association with R subunits analysed by co-IP. Cells were transfected with FLAG-tagged RIIβ (RIIβ-FLAG) and either wild-type (WT) or mutant Cα subunits. Shown are representative western blot analyses of Cα and RIIβ after FLAG-tagged RIIβ was immunoprecipitated with a FLAG-specific antibody (IP: FLAG). The western blot analyses in the lower part of the figure (input) control for expression levels of wild-type or mutant Cα and RIIβ. These analyses were repeated in at least six independent experiments with similar results. Full size image To further analyze the interaction between PKA Cα mutants and R subunits, we devised a second approach that monitored the basal association between the R and C subunits as well as their dissociation during a stepwise increase of the cAMP concentration. For this purpose, we took advantage of the well-known strong interaction of R subunits, but not of free C subunits, to anion exchange matrices, such as DEAE-Sephacel [20] . We allowed PKA from lysates of cells co-transfected with RIIβ and either wild-type or mutant Cα subunits to bind to DEAE-Sephacel. Then, we loaded the samples into small chromatography columns, eluted the columns with stepwise increasing concentrations of cAMP and measured both the amount of eluted Cα subunit (by western blot analysis) and PKA catalytic activity (using a gel-based assay) in the collected fractions. When lysates from cells co-transfected with wild-type Cα and RIIβ subunits were analysed, very little Cα subunit was found in the flow-through and initial washes (indicating strong binding), and an elution peak of the Cα subunit was observed at ~2 μM cAMP ( Fig. 3a ), consistent with the affinity of cAMP for the PKA holoenzyme [21] . This corresponded well to a peak in PKA activity ( Fig. 3b ). In contrast, when the wild-type Cα subunit was replaced by either mutant, PKA activity and the Cα subunit were recovered to a much larger extent already in the flow-through and/or wash fractions ( Fig. 3a–c ), suggesting that at most only a weak interaction between the Cα mutants and wild-type R subunits was present. 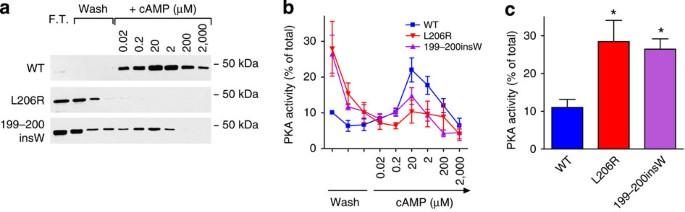Figure 3: Effect of Leu206Arg and Leu199_Cys200insTrp mutations on the retention of Cα subunits on DEAE-Sephacel. (a–c) Results of experiments where the lysates of cells co-transfected with R and C subunits were pre-bound to DEAE-Sephacel columns, which have a high affinity for R subunits, and eluted with wash buffer followed by the same buffer containing increasing concentrations of cAMP. Data are from 4 independent experiments per condition. (a) Western blot analysis for Cα. Shown are three representative blots. (b) PKA activity (mean±s.e.m.) measured in the different fractions (n=4). (c) Comparison of the fraction of PKA activity (mean±s.e.m.) collected during the first two washes with buffer (n=4). *P<0.05 versus WT by one-way ANOVA followed by Bonferroni’spost-hoctest. Figure 3: Effect of Leu206Arg and Leu199_Cys200insTrp mutations on the retention of Cα subunits on DEAE-Sephacel. ( a – c ) Results of experiments where the lysates of cells co-transfected with R and C subunits were pre-bound to DEAE-Sephacel columns, which have a high affinity for R subunits, and eluted with wash buffer followed by the same buffer containing increasing concentrations of cAMP. Data are from 4 independent experiments per condition. ( a ) Western blot analysis for Cα. Shown are three representative blots. ( b ) PKA activity (mean±s.e.m.) measured in the different fractions ( n =4). ( c ) Comparison of the fraction of PKA activity (mean±s.e.m.) collected during the first two washes with buffer ( n =4). * P <0.05 versus WT by one-way ANOVA followed by Bonferroni’s post-hoc test. Full size image In addition, we used a well-established assay based on FRET between cyan fluorescent protein (CFP)-tagged R and yellow fluorescent protein (YFP)-tagged C subunits [22] , [23] to monitor the cAMP-induced dissociation of the PKA holoenzyme ( Fig. 4a ). This assay was performed on cell lysates of Cos-7 cells that had been co-transfected with wild-type or mutant Cα and either a type-I (RIα) or a type-II (RIIβ) regulatory subunit. Addition of cAMP to lysates containing wild-type CFP-RIIβ and YFP-Cα subunits caused a rapid decrease in FRET, indicating that the C and R subunits were dissociating ( Fig. 4b,d ). In contrast, no change in FRET was observed when the same experiment was performed with either Cα mutant ( Fig. 4c,d ). Similar results were obtained when RIα was used instead of RIIβ ( Fig. 4e ). 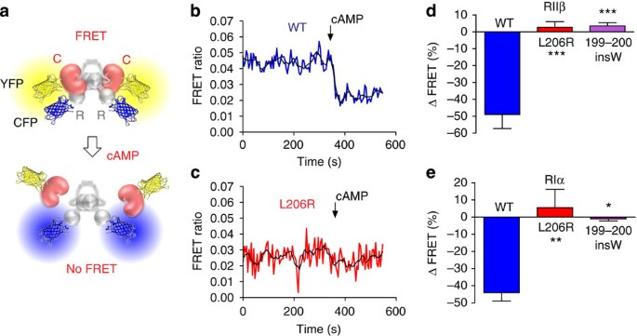Figure 4: Effect of Leu206Arg and Leu199_Cys200insTrp mutations on cAMP-dependent PKA dissociation. (a) Schematic representation of the fluorescently labelled PKA holoenzyme. In the absence of cAMP, FRET occurs between CFP attached to the R subunits and YFP attached to the C subunits, resulting in high YFP and low CFP emission. On cAMP binding to the R subunits and dissociation of the C subunits, FRET drops, leading to high CFP and low YFP emission. (b,c) Representative FRET traces obtained in lysates from cells transfected with RIIβ together with either wild-type Cα (b) or the Leu206Arg mutant (c). cAMP addition causes a robust drop of FRET in the presence of wild-type Cα (b) but not in the presence of the Leu206Arg mutant (c). The black traces were obtained by smoothing the data using a moving average of 13 neighbouring data points. (d,e) Comparison of the changes in FRET ratio (mean±s.e.m.) caused by cAMP addition among wild-type (WT) and mutant Cα co-expressed with either RIIβ (d) or RIα (e) subunits (n=4 for WT Cα and Leu199_Cys200insTrp mutant,n=5 for Leu206Arg mutant). Data are from at least four independent experiments per condition. *P<0.05 versus WT, **P<0.01 versus WT, ***P<0.001 versus WT by one-way ANOVA followed by Bonferroni’spost-hoctest. Figure 4: Effect of Leu206Arg and Leu199_Cys200insTrp mutations on cAMP-dependent PKA dissociation. ( a ) Schematic representation of the fluorescently labelled PKA holoenzyme. In the absence of cAMP, FRET occurs between CFP attached to the R subunits and YFP attached to the C subunits, resulting in high YFP and low CFP emission. On cAMP binding to the R subunits and dissociation of the C subunits, FRET drops, leading to high CFP and low YFP emission. ( b , c ) Representative FRET traces obtained in lysates from cells transfected with RIIβ together with either wild-type Cα ( b ) or the Leu206Arg mutant ( c ). cAMP addition causes a robust drop of FRET in the presence of wild-type Cα ( b ) but not in the presence of the Leu206Arg mutant ( c ). The black traces were obtained by smoothing the data using a moving average of 13 neighbouring data points. ( d , e ) Comparison of the changes in FRET ratio (mean±s.e.m.) caused by cAMP addition among wild-type (WT) and mutant Cα co-expressed with either RIIβ ( d ) or RIα ( e ) subunits ( n =4 for WT Cα and Leu199_Cys200insTrp mutant, n =5 for Leu206Arg mutant). Data are from at least four independent experiments per condition. * P <0.05 versus WT, ** P <0.01 versus WT, *** P <0.001 versus WT by one-way ANOVA followed by Bonferroni’s post-hoc test. Full size image To assess potential effects of the Cα mutations on PKA catalytic activity, we compared the PKA activity of cell lysates containing either wild-type or mutant Cα subunits in the presence of a saturating concentration of cAMP. For this purpose, we overexpressed tagged Cα and RIIβ subunits and correlated the cAMP-stimulated PKA activity in the cell lysates with the expression levels of the exogenous Cα subunits, using four different amounts of samples ( Fig. 5 ). No statistically significant differences were observed among the two mutants and the wild-type Cα subunit. These data indicate that the maximal activity (that is, the one measured in the presence of saturating cAMP concentrations) of both Cα mutants did not differ from that of the wild-type Cα subunit. 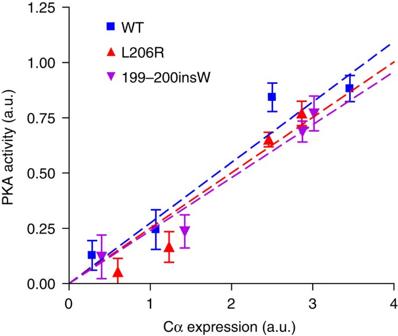Figure 5: Effect of Leu206Arg and Leu199_Cys200insTrp mutations on catalytic activity. Cells were transfected with wild-type or mutant Cα subunits tagged with YFP together with the CFP-tagged RIIβ subunit. Four different amounts of cells lysates were used. The PKA catalytic activity was measured in the presence of a saturating concentration of cAMP (200 μM). The amount of exogenous Cα subunits was quantified using an antibody that recognizes YFP. Shown are the results (mean±s.e.m.) of three independent measurements. Data were fit by linear regression. Differences among slopes are not statistically significant by an F-test. Figure 5: Effect of Leu206Arg and Leu199_Cys200insTrp mutations on catalytic activity. Cells were transfected with wild-type or mutant Cα subunits tagged with YFP together with the CFP-tagged RIIβ subunit. Four different amounts of cells lysates were used. The PKA catalytic activity was measured in the presence of a saturating concentration of cAMP (200 μM). The amount of exogenous Cα subunits was quantified using an antibody that recognizes YFP. Shown are the results (mean±s.e.m.) of three independent measurements. Data were fit by linear regression. Differences among slopes are not statistically significant by an F-test. Full size image Functional assessment of PKA Cα mutants in living cells Our in vitro results provided strong evidence that both mutations in the Cα subunit interfered with the formation of a stable PKA holoenzyme. To prove that the same was occurring also in intact cells, we performed a series of live-cell experiments in which we monitored the association between fluorescently tagged PKA subunits by means of FRET microscopy. To begin with, we assessed the basal interaction between PKA Cα mutants and R subunits by acceptor photobleaching. Whereas this method was able to detect an interaction between wild-type Cα and RIIβ subunits, no statistically significant interactions were measured in case of both Cα mutants ( Fig. 6a ). Then, we monitored in real-time FRET between PKA Cα mutants and R subunits in cells that were stimulated with a pharmacological activator of adenylyl cyclase (forskolin) to increase intracellular cAMP concentrations. Whereas a large decrease in FRET, indicative of PKA dissociation, was detected in the presence of wild-type Cα, virtually no changes were observed in the case of either Cα mutant ( Fig. 6b ). 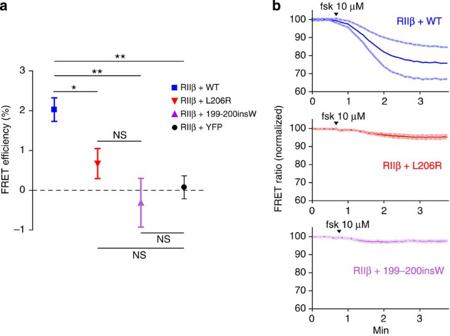Figure 6: FRET measurements in living cells. Cells were transfected with wild-type or mutant Cα subunits tagged with YFP together with the CFP-tagged RIIβ subunit. (a) Basal association of Leu206Arg and Leu199_Cys200insTrp mutants with RIIβ in living cells as measured by acceptor photobleaching FRET. Data (mean±s.e.m.) are taken from more than 90 cells analysed in six independent experiments for each condition. *P<0.05, **P<0.001; NS, statistically not significant by one-way ANOVA followed by Bonferroni’spost-hoctest. (b) Effect of increasing intracellular cAMP concentrations with forskolin (fsk, 10 μM) on the association between CFP-tagged RIIβ and either wild-type or mutant Cα subunits tagged with YFP. Data (mean±s.e.m.) are taken from 9 to 16 cells per condition measured in three independent experiments. Figure 6: FRET measurements in living cells. Cells were transfected with wild-type or mutant Cα subunits tagged with YFP together with the CFP-tagged RIIβ subunit. ( a ) Basal association of Leu206Arg and Leu199_Cys200insTrp mutants with RIIβ in living cells as measured by acceptor photobleaching FRET. Data (mean±s.e.m.) are taken from more than 90 cells analysed in six independent experiments for each condition. * P <0.05, ** P <0.001; NS, statistically not significant by one-way ANOVA followed by Bonferroni’s post-hoc test. ( b ) Effect of increasing intracellular cAMP concentrations with forskolin (fsk, 10 μM) on the association between CFP-tagged RIIβ and either wild-type or mutant Cα subunits tagged with YFP. Data (mean±s.e.m.) are taken from 9 to 16 cells per condition measured in three independent experiments. Full size image Taken together, these data indicate that both PKA Cα mutants identified in cortisol-secreting adrenal adenomas have normal enzymatic activity, but are unable to form a stable complex with R subunits both in vitro and in living cells, thus providing an explanation for their high constitutive activity and the loss of regulation by cAMP. This study provides a molecular basis to explain the pathogenic role of PRKACA mutations, which we have previously found to be frequently present in cortisol-secreting adrenal adenomas [13] . Our findings indicate that both mutations found in our previous study (Leu206Arg and Leu199_Cys200insTrp) interfere with the formation of a stable PKA holoenzyme, thus rendering the mutant PKA Cα subunits constitutively active. Very recent whole-exome-sequencing studies have confirmed the high frequency of the PRKACA variant Leu206Arg in cortisol-secreting adrenal adenomas [14] , [15] , [16] . These studies found an increased phosphorylation of PKA substrates in the presence of the Leu206Arg variant, in agreement with our previous findings [13] . However, the mechanism of action of the Leu206Arg mutation is highly controversial. On the basis of the finding that the Leu206Arg variant co-immunoprecipitated with R subunits, as well as of a higher basal PKA activity in cells co-transfected with the Leu206Arg variant and R subunits compared with cells co-transfected with wild-type Cα and R subunits, Cao et al. [14] concluded that the interaction of the Leu206Arg variant with R subunits is preserved. To explain their findings, they hypothesized that the Leu206Arg mutation might increase PKA activity by enhancing substrate interaction and/or the catalytic activity of the enzyme [14] . In contrast, two other studies [15] , [16] did not detect any co-IP between the Leu206Arg variant and RIα. Our study provides a direct measurement of the association of Leu206Arg and Leu199_Cys200insTrp mutants with R subunits under basal conditions and after cAMP stimulation both in vitro and in intact cells. Our results clearly indicate the presence of a major defect in this association for both Cα mutants, which is already observable in the absence of cAMP. These findings are consistent with the virtual lack of regulation by an excess of R subunits or by cAMP [13] . Whereas we cannot exclude that either mutation might also have an impact on substrate specificity, we did not observe a difference in the PKA activity (measured with Kemptide as a substrate) of samples containing either wild-type or mutant Cα in the presence of a saturating concentration of cAMP. Taken together, these data provide a molecular explanation for the increased PKA activity in cells harbouring either mutation identified in our previous study. The zona fasciculata of the adrenal cortex, which is responsible for glucocorticoid production, is under the strict control of the adrenocorticotropic hormone (ACTH) [24] . ACTH activates a G-protein-coupled receptor located on the surface of adrenocortical cells, which induces both cortisol production and cell proliferation through activation of the cAMP/PKA pathway [25] , [26] , [27] . Thus, a constitutive activation of PKA, as seen in the presence of PRKACA -activating mutations, is expected to lead to deregulated cortisol production and increased cell replication, similarly to what is seen with PRKAR1A -inactivating and GNAS -activating mutations [5] , [6] , [7] , [8] . PRKACA -activating mutations appear to be responsible for Cushing’s syndrome, which, if not promptly recognized and effectively treated, is associated with high morbidity and mortality [28] . A better understanding of the molecular mechanisms at the basis of adrenal Cushing’s syndrome might thus allow improving its diagnosis and provide novel and more rational pharmacological therapies. In addition, given the essential role of PKA signalling in virtually all cells of our organism, similar pathological mechanisms might be implicated in other diseases of both endocrine and non-endocrine origin. Thus, our findings provide novel and essential information to understand the pathogenesis of cortisol-secreting adrenal tumours and possibly other PKA-pathies, which could have important clinical and pharmacological implications. In summary, our study indicates that both PRKACA mutations found in cortisol-secreting adrenal tumours affect a key region of the Cα subunit that is involved in interaction with the inhibitory sequence of the R subunits. Both mutations interfere with this interaction, and thus with the formation of a stable PKA holoenzyme. The resulting free mutant Cα subunits are active irrespective of the intracellular concentration of cAMP, which leads to constitutive PKA activation and phosphorylation of PKA targets. Nevertheless, the maximal catalytic activity of both Cα mutants is not altered. These findings provide a biochemical explanation for the increased PKA activity observed in adrenal tumours harbouring these PRKACA mutations and also a causal mechanism for the associated Cushing’s syndrome. Plasmids Plasmids encoding wild-type human RIα, RIIβ and Cα subunits were purchased from Origene. Mutations in the sequence coding for the Cα subunit were introduced by PCR as described [13] . The constructs were then subcloned into the pcDNA3 vector by standard procedures. Specifically, fragments containing the entire PKA subunit coding sequences were amplified by PCR using primers containing a KpnI site (RIIβ subunit) or HindIII (C and RIα subunits) at the 5′-end and a NotI site at the 3′-end and inserted between the KpnI (RIIβ subunit) or HindIII (C and RIα subunits) and NotI sites of pcDNA3. Plasmids encoding YFP-tagged human PKA Cα and CFP-tagged human RIIβ subunits were generated by replacing mouse subunits with human PKA subunits in the constructs originally described by Zaccolo et al. [23] Specifically, fragments containing the entire PKA subunit coding sequences without stop codon were amplified by PCR using primers containing a NotI site at the 5′-end and a ClaI site at the 3′-end and used to replace the mouse subunits contained between a NotI site and a ClaI site in the original vectors. Mutations were introduced by PCR following standard methods. For generating the plasmid encoding the FLAG-tagged RIIβ subunit, a fragment containing the entire coding sequence of the human RIIβ subunit was amplified by PCR with a forward primer containing the FLAG tag (amino-acid sequence DYKDDDDA) and a KpnI site at the 5′-end and a reverse primer containing a NotI site at the 3′-end. This fragment was subsequently inserted between the KpnI and NotI sites of pcDNA3. Cell culture and transfection HEK293 and Cos-7 cells were obtained from American Type Culture Collection. Cells were cultured in Dulbecco’s modified Eagle’s medium supplemented with 10% FCS, 0.1 mg ml −1 streptomycin and 100 U ml −1 penicillin at 37 °C and 5% (vol/vol) CO 2 . Cell culture reagents were from PAN-Biotech. Cos-7 cells were seeded at a density of 2.5 × 10 6 cells per well onto 15-cm Petri dishes and allowed to grow for 6 h, after which they were transfected with Fugene HD (Promega) according to the manufacturer’s protocol. HEK293 cells were seeded at a density of 1.2 × 10 6 cells per well onto 10-cm Petri dishes or 0.25 × 10 6 cells per well onto six-well plates containing 24-mm round glass coverslips and allowed to grow for 24 h, after which they were transfected with the Effectene transfection kit (Qiagen) according to the manufacturer’s protocol. Ratios of transfected R and C subunit DNA were optimized to favour association between C and R subunits [13] . All experiments were performed 48 h after transfection. Preparation of membrane-free cell lysates Cells were washed thrice with ice-cold phosphate-buffered saline, scraped from the plate and resuspended in 600 μl 5/2 buffer (5 mM Tris-HCl, 2 mM EDTA, pH 7.4). Thereafter, samples were homogenized using an Ultraturrax device for 20 s on ice and centrifuged at 100,000 g for 30 min at 4 °C to remove membranes. FRET measurements on cell lysates FRET measurements on membrane-free cell lysates were performed using a Perkin-Elmer LS50B fluorescence spectrometer. The excitation was set at 437±10 nm to excite CFP and at 490±10 nm to excite YFP. Dissociation of the PKA holoenzyme during addition of cAMP (final concentration=200 μM) was followed in real-time by monitoring CFP emission at 475±10 nm and YFP emission at 525±10 nm on CFP excitation at 437±10 nm. Separation of R and C subunits on DEAE-Sephacel columns Membrane-free cell lysates obtained from three 15-cm Petri dishes were mixed with 300 μl of a 1:1 DEAE-Sephacel slurry (GE Healthcare Life Sciences) in 5/2 buffer and incubated for 2 h at 4 °C under continuous rotation. Then, the samples containing DEAE-Sephacel were packed into mini spin columns. After centrifugation at 7,600 g for 1 min to remove the flow-through and three washes with 5/2 buffer, the columns were repeatedly eluted with increasing concentrations of cAMP, ranging from 20 nM to 2 mM. Each elution step was repeated twice. All procedures were performed at 4 °C. PKA activity assay PKA catalytic activity was measured using the PepTag non-radioactive cAMP-dependent protein kinase assay (Promega), which uses a fluorescent Kemptide peptide as substrate, following the manufacturer’s instructions. Images of the gels were acquired with a gel documentation system (Herolab) and analysed using the ImageJ software ( http://rsbweb.nih.gov/ij ). Co-immunoprecipitation Cells were lysed with a buffer containing 150 mM NaCl, 1 mM EDTA, 1 mM EGTA, 1% Triton X-100 and 20 mM Tris-HCl, pH 7.5, supplemented with protease inhibitors (Complete Mini, Roche). Lysates were centrifuged at 20,000 g for 10 min at 4 °C. Supernatants were transferred to a new vial and incubated with protein-A Sepharose for 2 h at 4 °C under continuous rotation. Protein-A Sepharose was either preincubated with a rabbit polyclonal anti-FLAG antibody (Sigma-Aldrich, # F7425) or without antibodies to control for unspecific binding of Cα to protein-A Sepharose (mock precipitation). Preincubations were performed overnight at 4 °C under continuous rotation. After the incubation of protein-A Sepharose with the cell lysates, samples were washed five times with lysis buffer. Proteins were removed from protein-A Sepharose by addition of Laemmli buffer, followed by incubation for 3 min at 95 °C. Western blot analysis Unless otherwise indicated, samples were mixed with Laemmli buffer and incubated for 2 min at 95 °C. Proteins were separated by electrophoresis on a 10% SDS polyacrylamide gel and electrotransferred to a polyvinylidene difluoride membrane (Merck Millipore). Membranes were blocked with TBS-T (Tris-buffered saline with Tween 20) buffer+5% milk for 2 h at room temperature and incubated overnight at 4 °C with the indicated primary antibody, followed by incubation with an appropriate horseradish peroxidase-conjugated secondary antibody for 1 h at room temperature. PKA Cα subunits were detected with a rabbit polyclonal antibody (Cell Signaling # 4782, 1:5,000 dilution) or with a mouse monoclonal antibody (BD Transduction Laboratories # 610980, 1:4,000 dilution). YFP-tagged Cα subunits were detected using a rabbit polyclonal antibody against green fluorescent protein (Invitrogen # A6455, 1:1,000 dilution). FLAG-tagged RIIβ subunits were detected using a mouse monoclonal anti-FLAG antibody (Sigma-Aldrich # F3165, 1:8,000 dilution). Uncropped scans of western blots are given in Supplementary Fig. 2 . FRET measurements in living cells Imaging was performed in a buffer containing 144 mM NaCl, 5.4 mM KCl, 2 mM CaCl 2 , 1 mM MgCl 2 and 10 mM HEPES, pH 7.3. Ratiometric FRET experiments were performed on a Zeiss Axiovert 200 inverted microscope equipped with a × 63 oil-immersion objective, a polychrome V light source (Till Photonics), a 505 DCXR beam splitter and a CoolSNAP HQ CCD Camera (Photometrics). Images were acquired every 5 s with 5-ms illumination time and monitored with the MetaFluor 5.0 software (Molecular Devices) as the ratio between emission at 535±20 nm (YFP) and emission at 480±15 nm (CFP), on excitation at 436±10 nm. The YFP emission was corrected for direct excitation of YFP at 436 nm and the bleedthrough of CFP emission into the YFP channel. Acceptor photobleaching experiments were performed on a TCS SP5 confocal microscope (Leica Microsystems) using a × 63 oil-immersion objective. CFP was excited using the 458-nm line of a 65-mW argon-ion laser. CFP emission was detected with a GaAsP hybrid detector in a range from 465 to 490 nm. YFP bleaching was performed using the 514-nm line of the same laser set at 50%. To measure acceptor photobleaching, two separate CFP images were acquired, one before and one after YFP photobleaching. Images were analysed using the ImageJ software. After subtracting the background, FRET efficiency ( E ) was calculated from these images using the following equation [29] : where I 0 is the CFP intensity before and I bl is the corresponding value after photobleaching. Structural analysis of human mutations Structural images were prepared using the PyMOL software ( www.pymol.org ). The structure of the mouse full-length tetrameric RIIβ(2):Cα(2) holoenzyme [19] (Protein Data Bank entry 3TNP) was used to display the PKA catalytic (Cα) and regulatory (RIIβ) subunit structures. Statistical analyses Statistical analyses were performed using Prism 4.0 (GraphPad). Values are given as mean±s.e.m. Differences between three or more groups were assessed by one-way ANOVA followed by Bonferroni’s post-hoc test. Differences were considered significant for values of P <0.05. How to cite this article: Calebiro, D. et al. PKA catalytic subunit mutations in adrenocortical Cushing’s adenoma impair association with the regulatory subunit. Nat. Commun. 5:5680 doi: 10.1038/ncomms6680 (2014).